The Wnt3a/β-catenin target geneMesogenin1controls the segmentation clock by activating a Notch signalling program Segmentation is an organizing principle of body plans. The segmentation clock, a molecular oscillator best illustrated by the cyclic expression of Notch signalling genes, controls the periodic cleavage of somites from unsegmented presomitic mesoderm during vertebrate segmentation. Wnt3a controls the spatiotemporal expression of cyclic Notch genes; however, the underlying mechanisms remain obscure. Here we show by transcriptional profiling of Wnt3a −/− embryos that the bHLH transcription factor, Mesogenin1 (Msgn1) , is a direct target gene of Wnt3a. To identify Msgn1 targets, we conducted genome-wide studies of Msgn1 activity in embryonic stem cells. We show that Msgn1 is a major transcriptional activator of a Notch signalling program and synergizes with Notch to trigger clock gene expression. Msgn1 also indirectly regulates cyclic genes in the Fgf and Wnt pathways. Thus, Msgn1 is a central component of a transcriptional cascade that translates a spatial Wnt3a gradient into a temporal pattern of clock gene expression. Somites are blocks of paraxial mesoderm that bud from the anterior end of the presomitic mesoderm (PSM) every 2 h in the mouse embryo, and ultimately give rise to the musculoskeletal system. The timing of somitogenesis is controlled by a network of oscillating genes in the Notch, Wnt and Fgf signalling pathways [1] . Notch target genes such as Lunatic fringe ( Lfng ) are amongst the first cyclic genes to be characterized [2] . Lfng is first expressed in the posterior PSM and sweeps anteriorly, arresting as a stripe in the anterior PSM, before a repetitive wave of gene expression begins anew [3] , [4] , [5] . The oscillation frequency matches the rate of somite formation, leading to the proposal that cyclically expressed genes constitute a segmentation clock that controls the timing of somitogenesis [6] . The demonstration that the Notch/Fgf pathways oscillate out of phase with the Wnt pathway [1] , and that the loss of activity of any one of the signalling pathways adversely affects oscillatory gene expression in all three pathways [7] , [8] , [9] , [10] , strongly suggests that these signalling pathways interact in a coordinated and reciprocal fashion. Wnt3a, signalling via β-catenin, controls oscillatory gene expression in the Notch pathway since cyclic Lfng expression ceases in the absence of either gene [7] , [8] , [11] . Although it has been proposed that Wnt signalling does so through the direct activation of the Notch ligand Dll1 (ref. 12 ), Dll1 levels remain surprisingly robust in Wnt3a mutants despite the dramatic downregulation of other direct Wnt target genes such as Axin2 (refs 7 , 11 ). These results suggest that alternative mechanisms might account for the regulation of the Notch pathway and the segmentation clock by Wnt3a. A decreasing posterior–anterior gradient of Wnt3a/β-catenin and Fgf activity across the PSM has an important role in translating the rhythmic output of the segmentation clock into a periodic array of somites [7] , [13] . The Wnt/Fgf gradient positions segment boundaries by establishing a threshold of activity (termed the determination front), below which anterior PSM cells can respond to the segmentation clock by activating the boundary determination genes Mesoderm posterior 2 ( Mesp2 ) and Ripply2 (refs 8 , 14 , 15 , 16 ). Reduced Wnt3a/β-catenin signalling in the anterior PSM is crucial for determination front activity because the overactivation of β-catenin in the anterior PSM maintained the clock and blocked Mesp2 / Ripply2 expression, resulting in a profound elongation of the PSM and delayed somitogenesis [8] , [17] . Thus, Wnt3a functions in both the clock and the determination front during somitogenesis; however, it remains unclear how Wnt3a performs both functions. Stimulation of the Wnt/β-catenin signalling pathway stabilizes β-catenin, which interacts with members of the Lef/Tcf family of DNA-binding factors to activate the transcription of target genes [18] . We show here that the bHLH transcription factor gene Msgn1 is a target of the Wnt3a/β-catenin pathway and that the Wnt3a gradient defines the oscillatory field through the induction of Msgn1 . Msgn1 , in turn, directly activates the expression of Notch pathway genes, including cyclic genes. Thus, Msgn1 directly links the Wnt3a signalling gradient to the Notch signalling pathway and the segmentation clock. A Wnt3a gradient defines the Msgn1 spatial expression domain Transcriptional profiling of presomite-stage wildtype and Wnt3a −/− embryos revealed that Msgn1 is downregulated in Wnt3a mutants ( Fig. 1a ). Msgn1 was of particular interest since the Msgn1 −/− phenotype, which includes the absence of posterior somites [19] , is similar to the phenotypes observed in Wnt3a −/− and Ctnnb1 fl (β-catenin) mutants [8] , [20] . Msgn1 is an excellent candidate target gene of Wnt3a as it is spatiotemporally co-expressed with Wnt3a in the gastrulating ( Fig. 1b,c ) and segmenting ( Fig. 1d ) embryo. The Msgn1 anterior border lies posterior to the stripes of Mesp2/Ripply2 expression [21] and thus coincides with the position of the determination front. Importantly, the anteroposterior position of this border in the PSM depends on Wnt3a and Ctnnb1 activity. Wnt3a or Ctnnb1 loss-of-function (LOF) leads to a loss of Msgn1 expression ( Fig. 1e,f ), whereas the conditional stabilization of β-catenin in the PSM results in a remarkable anterior expansion of Msgn1 expression ( Fig. 1g ). To test if Wnt3a can activate Msgn1 dose-dependently, we treated pluripotent embryonic stem cells (ESC), which retain the potential to form mesoderm, with recombinant Wnt3a in serum-free conditions [22] . Wnt3a treatment led to a potent dose-dependent induction of Msgn1 messenger RNA ( Fig. 1h ). Taken together, the data suggest that the Wnt3a gradient spatially defines the Msgn1 expression domain in the PSM, and that the anterior border of Msgn1 may be an important component of the determination front. 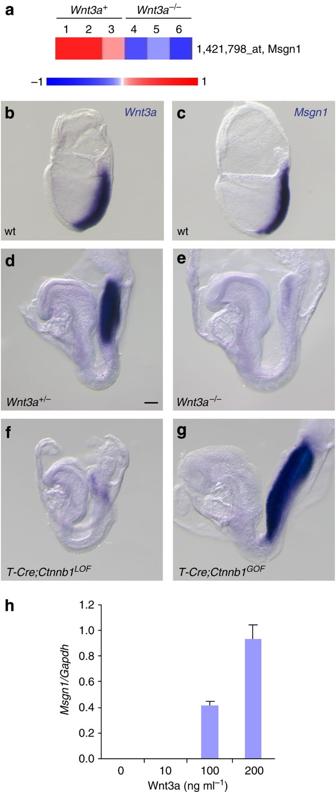Figure 1:Msgn1lies downstream of Wnt3a/β-catenin signalling. (a) Hierarchical clustering was used to visualize differences inMsgn1expression between E7.75–8 wildtype andWnt3a−/−embryos (P≤0.05, F-test) as detected by Affymetrix microarrays. Each column represents a pool of three stage-matched embryos. Upregulated (red) and downregulated (blue) gene expression is shown, with the magnitude of change reflected by the colour intensity. Colour scale bar represents log intensity values. (b,c) WISH analysis ofWnt3aexpression in the PS ectoderm (b), andMsgn1expression in the adjacent PS mesoderm (c), of E7.5 wildtype embryos. (d–g) WISH analysis ofMsgn1expression in the posterior PSM ofWnt3a+/−(d),Wnt3a−/−(e),T-Cre; Ctnnb1LOF(f),T-Cre;Ctnnb1GOF(g) embryos at E8.5. Note thatMsgn1expression in the posterior PSM defines the oscillatory field. (h) qPCR analysis ofMsgn1expression, normalized toGapdhlevels, in GFP-Bry ESC treated with recombinantWnt3ain serum-free conditions. Error bars represent standard deviation of 3 samples. GOF, gain of function. Scale bar, 100 μm. Figure 1: Msgn1 lies downstream of Wnt3a/β-catenin signalling. ( a ) Hierarchical clustering was used to visualize differences in Msgn1 expression between E7.75–8 wildtype and Wnt3a −/− embryos ( P ≤0.05, F-test) as detected by Affymetrix microarrays. Each column represents a pool of three stage-matched embryos. Upregulated (red) and downregulated (blue) gene expression is shown, with the magnitude of change reflected by the colour intensity. Colour scale bar represents log intensity values. ( b , c ) WISH analysis of Wnt3a expression in the PS ectoderm ( b ), and Msgn1 expression in the adjacent PS mesoderm ( c ), of E7.5 wildtype embryos. ( d – g ) WISH analysis of Msgn1 expression in the posterior PSM of Wnt3a +/− ( d ), Wnt3a −/− ( e ), T-Cre; Ctnnb1 LOF ( f ), T-Cre ; Ctnnb1 GOF ( g ) embryos at E8.5. Note that Msgn1 expression in the posterior PSM defines the oscillatory field. ( h ) qPCR analysis of Msgn1 expression, normalized to Gapdh levels, in GFP-Bry ESC treated with recombinant Wnt3a in serum-free conditions. Error bars represent standard deviation of 3 samples. GOF, gain of function. Scale bar, 100 μm. Full size image Although our genetic studies, together with in vitro and transgenic analyses of the Msgn1 promoter ( Fig. 2a–d ), clearly demonstrate that Msgn1 is directly controlled by a Wnt3a signalling gradient, Msgn1 is not highly graded across the PSM at early somitogenesis stages ( Fig. 1d ) suggesting that additional regulators maintain Msgn1 in more rostral domains. Previous analysis of the Msgn1 promoter showed that Msgn1 is activated by the Tbox transcription factor Tbx6, in addition to Wnt signalling [23] . Tbx6 is another important regulator of somitogenesis [24] and is thought to be expressed in an identical domain as Msgn1 (ref. 21 ). Re-examination of Tbx6 and Msgn1 co-expression demonstrates that although similar, Tbx6 expression exceeds Msgn1 ( Fig. 2e,f ), suggesting that Tbx6 is insufficient to define the position of the Msgn1 anterior border. To determine whether Tbx6 is required for Msgn1 expression in the anterior PSM, we examined (embryonic day) E8.5 Tbx6 −/− embryos by whole-mount in situ hybridization (WISH) and found that the anterior border of the Msgn1 domain was indeed shifted posteriorly, and Msgn1 mRNA was now expressed in a graded fashion in the posterior-most PSM ( Fig. 2g,h ). Reducing Wnt3a dosage on the Tbx6 −/− background led to reductions in Msgn1 expression below levels observed in Tbx6 −/− embryos ( Supplementary Fig. S1 ), providing genetic evidence that the weak, graded Msgn1 expression observed in Tbx6 mutants depends upon Wnt3a. We conclude that Tbx6 maintains Msgn1 expression in the anterior PSM, functioning together with a Wnt3a gradient to generate an anterior boundary that defines the determination front. 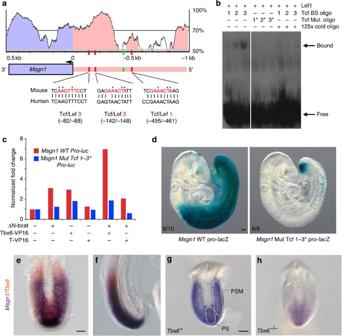Figure 2:Msgn1is directly activated by the Wnt/β-catenin pathway and Tbx6. (a) VISTA 'peaks and valleys' plot57illustrating a comparative analysis of the mouse and humanMsgn1loci (blue) including 1 kb of the upstream regulatory region (pink). The percent of conservation (yaxis) between the two organisms is plotted against the coordinates of the mouse sequence (xaxis). The pink regions are conserved non-coding regions, and the blue region is the conservedMsgn1exon. The position of conserved consensus Tcf/Lef (red bars) and Tbox (green bar) binding sites identified in the promoter are displayed below the VISTA plot. Asterisks indicate nucleotides mutated for EMSA and transgenic reporter assays. (b) EMSA assay demonstrating the specific binding of Lef1 protein to Tcf/Lef BS probes but not to probes carrying mutated Tcf/Lef sites (asterisks). Lef1 binding to wild-type probes is competed by the addition of 125 times excess unlabelled probe. (c) Luciferase reporter assays for 1 kb of the mouseMsgn1promoter. Transfection of 293 cells with ΔN-β-catenin, orTbx6-VP16 alone moderately activated the wild-type 1 kbMsgn1promoter, whereas co-transfection of both ΔN-β-catenin andTbx6-VP16 resulted in a 7-fold activation. Co-expression of T-VP16 with ΔN-β-catenin did not result in a similar effect. Point mutations in all three Tcf/Lef BS abolished the activation of the luciferase reporter byTbx6-VP16 and/or ΔN-β-catenin. (d) Representative transient transgenic embryos expressing the 1 kb wildtypeMsgn1promoter-lacZreporter (left) or a mutant version carrying mutations in all three Tcf/Lef BS (right). The fraction (bottom left corner) represents the number of embryos displaying the demonstrated pattern/total number of βgal positive transgenic founders. (e,f) 2 colour WISH ofMsgn1(purple) andTbx6(orange) co-expression in E9 PSM, (e,f) are dorsal and lateral views, respectively.Tbx6expression extends beyond the anterior border ofMsgn1expression. (g,h) Dorsal-posterior views ofMsgn1mRNA in E8.5 wild-type littermate controls (g) andTbx6−/−(h) embryos, oriented with posterior pointing down. Abbr.: BS, binding site. GOF, gain of function. Scale bar, 100 μm. Figure 2: Msgn1 is directly activated by the Wnt/β-catenin pathway and Tbx6. ( a ) VISTA 'peaks and valleys' plot [57] illustrating a comparative analysis of the mouse and human Msgn1 loci (blue) including 1 kb of the upstream regulatory region (pink). The percent of conservation ( y axis) between the two organisms is plotted against the coordinates of the mouse sequence ( x axis). The pink regions are conserved non-coding regions, and the blue region is the conserved Msgn1 exon. The position of conserved consensus Tcf/Lef (red bars) and Tbox (green bar) binding sites identified in the promoter are displayed below the VISTA plot. Asterisks indicate nucleotides mutated for EMSA and transgenic reporter assays. ( b ) EMSA assay demonstrating the specific binding of Lef1 protein to Tcf/Lef BS probes but not to probes carrying mutated Tcf/Lef sites (asterisks). Lef1 binding to wild-type probes is competed by the addition of 125 times excess unlabelled probe. ( c ) Luciferase reporter assays for 1 kb of the mouse Msgn1 promoter. Transfection of 293 cells with ΔN-β-catenin, or Tbx6 -VP16 alone moderately activated the wild-type 1 kb Msgn1 promoter, whereas co-transfection of both ΔN-β-catenin and Tbx6 -VP16 resulted in a 7-fold activation. Co-expression of T-VP16 with ΔN-β-catenin did not result in a similar effect. Point mutations in all three Tcf/Lef BS abolished the activation of the luciferase reporter by Tbx6 -VP16 and/or ΔN-β-catenin. ( d ) Representative transient transgenic embryos expressing the 1 kb wildtype Msgn1 promoter -lacZ reporter (left) or a mutant version carrying mutations in all three Tcf/Lef BS (right). The fraction (bottom left corner) represents the number of embryos displaying the demonstrated pattern/total number of βgal positive transgenic founders. ( e , f ) 2 colour WISH of Msgn1 (purple) and Tbx6 (orange) co-expression in E9 PSM, ( e , f ) are dorsal and lateral views, respectively. Tbx6 expression extends beyond the anterior border of Msgn1 expression. ( g , h ) Dorsal-posterior views of Msgn1 mRNA in E8.5 wild-type littermate controls ( g ) and Tbx6 −/− ( h ) embryos, oriented with posterior pointing down. Abbr. : BS, binding site. GOF, gain of function. Scale bar, 100 μm. Full size image Msgn1 functions in the clock and determination front The initial characterization of the segmentation phenotype in Msgn1 −/− embryos was performed at E9.5, a relatively late stage when mutants already lack posterior somites and PSM and display enlarged tailbuds [19] . The highly abnormal tailbud complicates the interpretation of the segmentation phenotype since the lack of posterior somites could be secondary to an inability of tailbud progenitors to migrate or give rise to PSM fates. Therefore, to address the potential role that Msgn1 may have in the determination front, we examined Msgn1 −/− mutants for the expression of the segment boundary determination genes Ripply2 and Mesp2 , and the posterior somite marker Uncx4.1 , at E8.5 when mutants are not clearly distinguished from littermates. WISH analysis revealed that all three genes were downregulated, whereas the primitive streak (PS) marker, Fgf8 , was unaffected ( Fig. 3 ). The lack of expression of segment boundary determination genes at early somitogenesis stages demonstrates that Msgn1 is required for determination front activity and suggests that Msgn1 is a functional effector of the Wnt3a gradient. 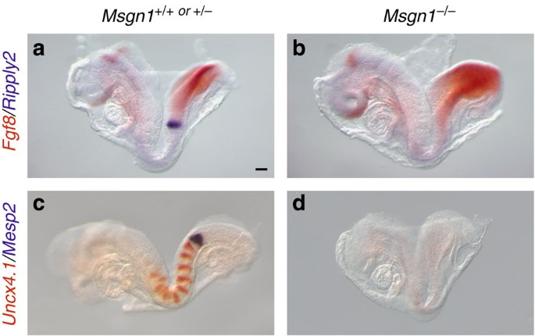Figure 3: Segment boundary determination genes are not expressed inMsgn1mutants. Two-colour WISH expression analysis of E8.5 wildtype (a,c), andMsgn1−/−(b,d) embryos for the expression ofFgf8(orange) andRipply2(purple) (a,b) andUncx4.1(orange) andMesp2(purple) (c,d). All views are lateral, and embryos are oriented with anterior to the left. Scale bar, 100 μm. Figure 3: Segment boundary determination genes are not expressed in Msgn1 mutants. Two-colour WISH expression analysis of E8.5 wildtype ( a , c ), and Msgn1 −/− ( b , d ) embryos for the expression of Fgf8 (orange) and Ripply2 (purple) ( a , b ) and Uncx4.1 (orange) and Mesp2 (purple) ( c , d ). All views are lateral, and embryos are oriented with anterior to the left. Scale bar, 100 μm. Full size image Msgn1 may also have an important role in the segmentation clock because cycling genes in the Notch pathway were shown to be downregulated in Msgn1 mutants at E9.5 (ref. 19 ). Because this reduced gene expression could arise secondarily, owing to the large number of apoptotic cells reported in the E9.5 Msgn1 −/− tailbud [19] , we reinvestigated the expression of cycling genes at the earlier E8.5 stage. We first examined mutants for the expression of cyclic Fgf and Wnt pathway genes, as interactions between all three signalling pathways are necessary for a functional segmentation clock. WISH analysis of Msgn1 −/− embryos, or explanted PSMs processed by the 'fix and culture' method [6] to assess the dynamic expression of cycling genes, revealed that the cyclic Wnt target genes Sp5 ( Fig. 4a–f ) and Axin2 (not shown) were upregulated and anteriorly expanded ( Fig. 4a,b ) but did not oscillate in the Msgn1 −/− PSM ( Fig. 4c–f ). The oscillating Fgf pathway genes Sprouty2 ( Fig. 4g–l ) and Dusp6 (not shown) were expressed at similar levels in mutants and controls ( Fig. 4g,h ), but cyclic expression was not observed in Msgn1 mutants either ( Fig. 4i–l ). Because all of the Wnt and Fgf target genes examined were expressed, we conclude that Msgn1 is not required for their activation. However, the static expression patterns in Msgn1 −/− explants after culture suggests that Msgn1 is required, directly or indirectly, for the oscillatory expression of cyclic Wnt and Fgf target genes. 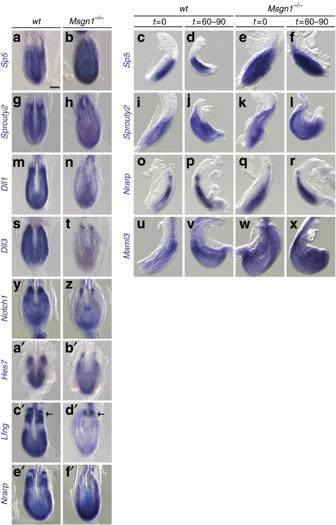Figure 4: Segmentation clock gene expression inMsgn1−/−mutants. WISH analysis ofSp5(a–f),Sprouty2(g–l),Dll1(m,n),Dll3(s,t),Notch1(y,z),Hes7(a′,b′),Lfng(c′,d′),Nrarp(e′,f′,o–r), andMaml3(u–x) expression in wildtype orMsgn1−/−embryos at E8.5. The cyclic Wnt target genesSp5(a) andAxin2(n=6, not shown) were upregulated in theMsgn1−/−PSM (n=4;b). (c–f) Lateral views of half-embryo explants analysed forSp5expression. Using the 'fix-and-culture' method, gene expression was assessed in a fixed, reference PSM explanted from one-half of a wild-type (wt) orMsgn1−/−embryo (t=0), and compared with its expression in the complementary half after culturing for roughly a half-cycle of cyclic gene expression (60–90 min). Spatially,Sp5expression in the wt PSM (c) changed after culture (d), indicative of dynamic oscillating expression, however, expression in theMsgn1−/−PSM was upregulated (n=2;e) and did not vary upon culture (f). The overall expression levels of the oscillating Fgf pathway genesSprouty2(g,h) andDusp6(n=4, not shown), did not change between wt (g) and mutant (n=5;h). Subtle variations inSprouty2expression in wt PSM explants before (i) and after (j) culture, were less apparent inMsgn1−/−PSM explants before (k) and after (l) culture. In contrast,Dll1was strongly expressed in the wt PSM (m) but was nearly absent in theMsgn1−/−PSM (n=5;n). Similarly,Dll3(n=5;s,t),Notch1(n=5;y,z),Hes7(n=5;a′,b′), andLfng(n=8;c′,d′) were significantly downregulated in theMsgn1−/−posterior PSM but weak expression persisted in the anterior PSM (arrows,c′,d′). AlthoughNrarp(e′) andMaml3(n=11; not shown) were strongly expressed in theMsgn1−/−posterior PSM (n=9;f′),Nrarpwas not expressed in stripes inMsgn1−/−embryos as it was in wild-type littermates, and expression was graded, more closely resembling Wnt target gene expression than Notch target genes (cf.4f′with4bandd′). Fix-and-culture experiments revealed that theNrarpspatial expression domain was dynamic in cultured wildtype explants (o,p) but did not change inMsgn1−/−explants (n=5;q,r). Similar results were observed forMaml3(n=2;u–x). Scale bar, 100 μm. Figure 4: Segmentation clock gene expression in Msgn1 −/− mutants. WISH analysis of Sp5 ( a – f ), Sprouty2 ( g – l ), Dll1 ( m , n ), Dll3 ( s , t ), Notch1 ( y , z ), Hes7 ( a′ , b′ ), Lfng ( c′ , d′ ), Nrarp ( e′ , f′ , o – r ), and Maml3 ( u – x ) expression in wildtype or Msgn1 −/− embryos at E8.5. The cyclic Wnt target genes Sp5 ( a ) and Axin2 ( n =6, not shown) were upregulated in the Msgn1 −/− PSM ( n =4; b ). ( c – f ) Lateral views of half-embryo explants analysed for Sp5 expression. Using the 'fix-and-culture' method, gene expression was assessed in a fixed, reference PSM explanted from one-half of a wild-type (wt) or Msgn1 −/− embryo ( t =0), and compared with its expression in the complementary half after culturing for roughly a half-cycle of cyclic gene expression (60–90 min). Spatially, Sp5 expression in the wt PSM ( c ) changed after culture ( d ), indicative of dynamic oscillating expression, however, expression in the Msgn1 −/− PSM was upregulated ( n =2; e ) and did not vary upon culture ( f ). The overall expression levels of the oscillating Fgf pathway genes Sprouty2 ( g , h ) and Dusp6 ( n =4, not shown), did not change between wt ( g ) and mutant ( n =5; h ). Subtle variations in Sprouty2 expression in wt PSM explants before ( i ) and after ( j ) culture, were less apparent in Msgn1 −/− PSM explants before ( k ) and after ( l ) culture. In contrast, Dll1 was strongly expressed in the wt PSM ( m ) but was nearly absent in the Msgn1 −/− PSM ( n =5; n ). Similarly, Dll3 ( n =5; s , t ), Notch1 ( n =5; y , z ), Hes7 ( n =5; a′ , b′ ), and Lfng ( n =8; c′ , d′ ) were significantly downregulated in the Msgn1 −/− posterior PSM but weak expression persisted in the anterior PSM (arrows, c′ , d′ ). Although Nrarp ( e′ ) and Maml3 ( n =11; not shown) were strongly expressed in the Msgn1 −/− posterior PSM ( n =9; f′ ), Nrarp was not expressed in stripes in Msgn1 −/− embryos as it was in wild-type littermates, and expression was graded, more closely resembling Wnt target gene expression than Notch target genes (cf. 4f′ with 4b and d′ ). Fix-and-culture experiments revealed that the Nrarp spatial expression domain was dynamic in cultured wildtype explants ( o , p ) but did not change in Msgn1 −/− explants ( n =5; q , r ). Similar results were observed for Maml3 ( n =2; u – x ). Scale bar, 100 μm. Full size image Although the cyclic Notch targets Lfng and Hes1 are not expressed in Msgn1 mutants at E9.5, Dll1 expression was reportedly reduced but not severely affected [19] , and other cyclic Notch genes such as Notch-regulated ankyrin-repeat protein ( Nrarp ) [25] , [26] , the Notch transcriptional coactivator Mastermind-like 3 ( Maml3 ) [27] , and the periodic transcriptional repressor Hes7 (ref. 28 ) were not examined. To determine whether Msgn1 has a central role in the regulation of known Notch clock genes, we examined their expression in Msgn1 −/− embryos at E8.5. WISH showed that numerous Notch pathway genes including Dll1 , Dll3 , Notch1 , Hes7, and Lfng were significantly downregulated in the posterior PSM ( Fig. 4m,n,s,t,y–d′ ). The Lfng expression pattern closely resembles the expression of Lfng in embryos lacking the transcriptional effector of the Notch pathway, RBP-JK [29] , [30] , suggesting that Msgn1 and RBP-JK have equivalent roles in Lfng regulation. In contrast, Nrarp ( Fig. 4e′,f′ ) and Maml3 (not shown) were strongly expressed in the posterior PSM of Msgn1 −/− embryos. Examination of cultured PSM explants demonstrated that the stripes of Nrarp expression in the control PSM ( Fig. 4o ) became broader in the posterior-most PSM of the complementary half after culture ( Fig. 4p ). In the Msgn1 −/− PSM, a large, graded, expression domain was observed ( Fig. 4q ), and this pattern remained unchanged after culture ( Fig. 4r ) indicating that Nrarp expression did not oscillate. Similarly, Maml3 was broadly expressed in Msgn1 −/− PSM, and the pattern remained unchanged after culture ( Fig. 4w,x ). These results demonstrate that neither Msgn1 , nor Notch signalling, is required for Nrarp and Maml3 activation, but Msgn1 is necessary for their cyclic expression. In summary, the expression of Dll1 , Dll3 , Notch1 , Hes7 and Lfng was dramatically reduced in the posterior PSM by the absence of Msgn1 , while Nrarp and Maml3 expression was qualitatively different. The lack of oscillatory expression of cyclic Notch, Wnt, and Fgf target genes indicate that Msgn1 plays a central and fundamental role in the segmentation clock. Genomic approaches to identify Msgn1 target genes To address the molecular mechanisms of Msgn1 function in the clock and gradient, we sought to identify the target genes of Msgn1 by genome-wide transcriptional profiling. Because early embryos provide extremely limiting amounts of tissue, ESC reagents were developed to exploit the ability of pluripotent ESC to self-renew indefinitely and to differentiate into mesoderm, including PSM, in vitro [22] . Recombinant ESC lines expressing a Doxycycline-inducible (Dox) FLAG epitope-tagged Msgn1 (F-Msgn1) ( Supplementary Fig. S2 ) [31] , were cultured in suspension for 2 days to initiate epiblast differentiation, and then induced with Dox to prematurely express Msgn1. Transcriptional profiles of embryoid bodies (EB)±F-Msgn1 induction were assessed for differentially expressed genes. Examination of the cyclic Wnt ( Sp5 and Axin2 ) and Fgf ( Spry2 and Dusp6 ) pathway genes revealed that ectopic Msgn1 expression had little effect on their expression ( Supplementary Fig. S3 ). Conversely, multiple genes in the Notch pathway were induced >1.5-fold by Msgn1, including Dll1 , Dll3 , Notch1 , and Nrarp ( Fig. 5a ; Supplementary Table S1 ). Differential Lfng expression was not statistically significant because of variable expression in both treated and untreated cells. Quantitative PCR (qPCR) analysis validated the microarray data for all Notch genes examined ( Fig. 5b ). Notably, Maml3 , which is not represented on the Affymetrix MOE430 2.0 gene chips, was also upregulated. Thus Msgn1 induced the expression of 6 different genes in the Notch signalling pathway. 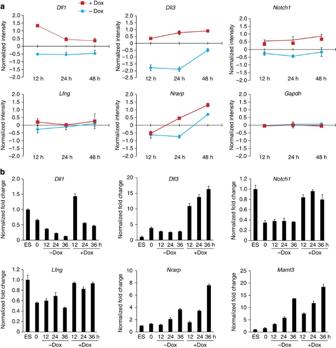Figure 5: Expression of Msgn1 in differentiating ESC rapidly induces Notch signalling genes. (a) Microarray analysis of gene expression in F-Msgn1 EBs in the absence (blue) and presence of Dox (red) over a 48-h timecourse. log2 ratios of the normalized expression levels ofDll1,Dll3,Notch1,Lfng,Nrarpand the housekeeping controlGapdhare presented.Lfngexpression was variable in Dox treated and untreated cells, presumably reflecting the dynamic expression of a cyclic gene, but was generally elevated by F-Msgn1 expression. Error bars indicate standard deviation of three biological replicates. (b) qPCR analysis of Notch pathway gene expression in F-Msgn1 ESC and EBs validates the microarray results shown in (a). Here error bars indicate standard deviation of 3 replicates. Figure 5: Expression of Msgn1 in differentiating ESC rapidly induces Notch signalling genes. ( a ) Microarray analysis of gene expression in F-Msgn1 EBs in the absence (blue) and presence of Dox (red) over a 48-h timecourse. log2 ratios of the normalized expression levels of Dll1 , Dll3 , Notch1 , Lfng , Nrarp and the housekeeping control Gapdh are presented. Lfng expression was variable in Dox treated and untreated cells, presumably reflecting the dynamic expression of a cyclic gene, but was generally elevated by F-Msgn1 expression. Error bars indicate standard deviation of three biological replicates. ( b ) qPCR analysis of Notch pathway gene expression in F-Msgn1 ESC and EBs validates the microarray results shown in ( a ). Here error bars indicate standard deviation of 3 replicates. Full size image The rapid activation of multiple Notch pathway genes suggests that Msgn1 could regulate their transcription directly. To determine whether Msgn1 binds to these loci, anti-Flag antibodies were used to immunoprecipitate chromatin bound to F-Msgn1, followed by sequencing (ChIP-seq) of F-Msgn1-associated DNA. Remarkably, multiple regions of the genome with significant enrichment in Msgn1-associated sequences were identified within, or upstream of, genes in the Notch pathway. Large Msgn1 peaks were found in conserved intronic regions of Notch1 , Notch2 , and Maml3 , and in upstream regulatory regions of Dll1 , Dll3 , Notch1 and Lfng ( Figs 6 and 7 ). Small Msgn1 peaks were also identified upstream of Dll1 ( Fig. 6a ), Nrarp and Sprouty2 , while none were associated with the Hes7 , Sp5 , Axin2 , or Dusp6 loci. Sequence analysis revealed the presence of at least one consensus E box motif (CANNTG) in each Msgn1 peak ( Fig. 6 ; Supplementary Fig. S4 ). As bHLH transcription factors bind to E boxes [32] , their presence is consistent with Msgn1 activating Notch pathway genes by direct binding. 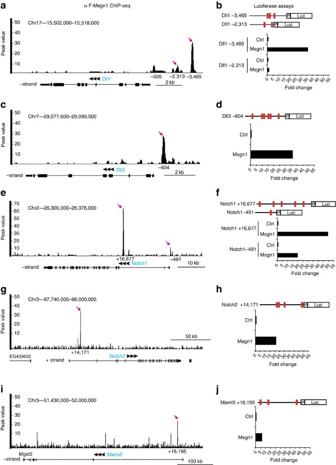Figure 6: F-Msgn1 binds directly to regulatory elements to transactivate multiple Notch pathway genes. F-Msgn1 immunoprecipitation in differentiating EBs enriches for chromatin at regulatory regions of Notch signalling genes such as the Notch ligandDll1(a). A strong peak at position −3,465, and a weak peak at position −2,313 (pink arrows) identify potential regulatory elements upstream of theDll1transcriptional start site. Theyaxis denotes the peak values. Peaks are numbered according to their position of the peak midpoint relative to the transcriptional start site. TheDll1locus is depicted below the peak map and the black arrowheads indicate orientation. Pink arrows indicate the specific enhancer elements tested for functional activity in luciferase reporter assays in NIH3T3 cells (b). Putative enhancer constructs are schematized at the top with red boxes indicating E-box consensus sequences. Luciferase reporter results are depicted as fold change.Dll1-3465 was strongly activated by Msgn1 expression (>35-fold) over the control expression vector (b) howeverDll1-2313 did not respond to Msgn1. Thus, functional enhancer activity strongly correlated with the strength of Msgn1 binding, as reflected by ChIP-seq peak values. A F-Msgn1 ChIP-seq peak inDll3(c) identified an upstream enhancer that drove strong Msgn1-dependent luciferase reporter expression (d). F-Msgn1 ChIP identified theNotch1promoter (−491) as well as a novel enhancer in the second intron (+16,677) (e), both of which were highly sensitive to Msgn1 activation (f). Similarly, enhancer elements that bound F-Msgn1, and that were activated by Msgn1 expression in reporter assays, were identified in the first intron ofNotch2(g,h) andMaml3(i,j). Figure 6: F-Msgn1 binds directly to regulatory elements to transactivate multiple Notch pathway genes. F-Msgn1 immunoprecipitation in differentiating EBs enriches for chromatin at regulatory regions of Notch signalling genes such as the Notch ligand Dll1 ( a ). A strong peak at position −3,465, and a weak peak at position −2,313 (pink arrows) identify potential regulatory elements upstream of the Dll1 transcriptional start site. The y axis denotes the peak values. Peaks are numbered according to their position of the peak midpoint relative to the transcriptional start site. The Dll1 locus is depicted below the peak map and the black arrowheads indicate orientation. Pink arrows indicate the specific enhancer elements tested for functional activity in luciferase reporter assays in NIH3T3 cells ( b ). Putative enhancer constructs are schematized at the top with red boxes indicating E-box consensus sequences. Luciferase reporter results are depicted as fold change. Dll1 -3465 was strongly activated by Msgn1 expression (>35-fold) over the control expression vector ( b ) however Dll1 -2313 did not respond to Msgn1. Thus, functional enhancer activity strongly correlated with the strength of Msgn1 binding, as reflected by ChIP-seq peak values. A F-Msgn1 ChIP-seq peak in Dll3 ( c ) identified an upstream enhancer that drove strong Msgn1-dependent luciferase reporter expression ( d) . F-Msgn1 ChIP identified the Notch1 promoter (−491) as well as a novel enhancer in the second intron (+16,677) ( e ), both of which were highly sensitive to Msgn1 activation ( f ). Similarly, enhancer elements that bound F-Msgn1, and that were activated by Msgn1 expression in reporter assays, were identified in the first intron of Notch2 ( g , h ) and Maml3 ( i , j ). 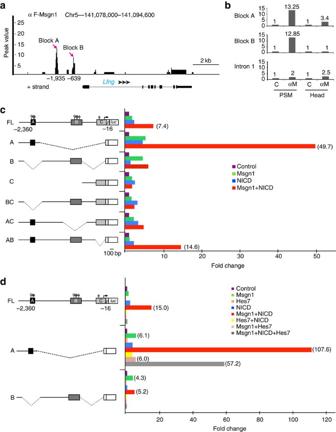Figure 7:Msgn1binds directly to clock enhancers in ESCs andin vivoand synergizes with Notch to activateLfng. (a) F-Msgn1 ChIP-seq peaks map to demonstrated clock enhancers in blocks A and B in the 5′ regulatory region ofLfngin differentiating EBs. Blocks A, B (and C) represent regions of sequence homology conserved between mouse and human30,33. (b) ChIP-qPCR analysis performed on PSMs or head tissue dissected from wild-type embryos demonstrates that endogenous Msgn1 binds strongly to Blocks A and B of theLfngenhancer in the PSM, relative to the head, and not to control regions in intron 1.yaxis represents fold change. C, control ascites fluid; αM, anti-Msgn1. (c)Lfng-luciferasereporter constructs containing up to 2.3 kb of theLfngenhancer/promoter are depicted on the left. Circles depict Rbpjk binding sites whereas triangles represent E-boxes. The luciferase activity for each construct, co-transfected with control (purple), Msgn1 (green), and/or activated Notch (NICD, blue) expression constructs in 3T3 cells is expressed as a fold change on the right. Msgn1 plus NICD (red) synergistically activate the full-length (FL) 2.3-kbLfngconstruct 7.4-fold, and the block A construct 49.7-fold. The A block is the only element capable of negotiating synergistic interactions between Msgn1 and NICD. (d) The cyclic transcriptional repressor Hes7 (orange) completely blocks the Msgn1/NICD synergism on the FL Lfng enhancer construct and requires the B block for maximal inhibitory activity. The combined activities of Hes7 with NICD (yellow), Hes7 and Msgn1 (pink), and Hes7 with Msgn1+NICD (grey) are illustrated. Full size image Figure 7: Msgn1 binds directly to clock enhancers in ESCs and in vivo and synergizes with Notch to activate Lfng . ( a ) F-Msgn1 ChIP-seq peaks map to demonstrated clock enhancers in blocks A and B in the 5′ regulatory region of Lfng in differentiating EBs. Blocks A, B (and C) represent regions of sequence homology conserved between mouse and human [30] , [33] . ( b ) ChIP-qPCR analysis performed on PSMs or head tissue dissected from wild-type embryos demonstrates that endogenous Msgn1 binds strongly to Blocks A and B of the Lfng enhancer in the PSM, relative to the head, and not to control regions in intron 1. y axis represents fold change. C, control ascites fluid; αM, anti-Msgn1. ( c ) Lfng-luciferase reporter constructs containing up to 2.3 kb of the Lfng enhancer/promoter are depicted on the left. Circles depict Rbpjk binding sites whereas triangles represent E-boxes. The luciferase activity for each construct, co-transfected with control (purple), Msgn1 (green), and/or activated Notch (NICD, blue) expression constructs in 3T3 cells is expressed as a fold change on the right. Msgn1 plus NICD (red) synergistically activate the full-length (FL) 2.3-kb Lfng construct 7.4-fold, and the block A construct 49.7-fold. The A block is the only element capable of negotiating synergistic interactions between Msgn1 and NICD. ( d ) The cyclic transcriptional repressor Hes7 (orange) completely blocks the Msgn1/NICD synergism on the FL Lfng enhancer construct and requires the B block for maximal inhibitory activity. The combined activities of Hes7 with NICD (yellow), Hes7 and Msgn1 (pink), and Hes7 with Msgn1+NICD (grey) are illustrated. Full size image Interestingly, the two Msgn1 peaks found in the Lfng locus precisely align with two previously described enhancers that drive Lfng expression in the PSM of transgenic embryos ( Fig. 7a [30] , [33] ). Peaks were also identified in the Dll1 and Dll3 loci that are distinct from, but overlapping with, previously defined regulatory elements [34] , [35] . To test these putative enhancers for Msgn1 responsiveness, peak sequences were cloned upstream of a minimal promoter driving the luciferase reporter and co-transfected with Msgn1 or control expression vectors in NIH3T3 cells. Msgn1 strongly transactivated the luciferase reporter in eight constructs (single peaks in Dll1 , Dll3 , Notch2 , and Maml3 ; and 2 peaks in Notch1 , and Lfng ( Figs 6b,d,f,h,j and 7c,d ). Two small ChIP-seq peaks, ( Dll1-505 and -2313 ) immediately upstream of the Dll1 transcriptional start site, were not found to be significantly different from control input DNA and thus were not scored as peaks. To verify that these sequences did not contain Msgn1 responsive elements, we tested one ( Dll1-2313 ) in reporter assays. Dll1-2313 did not respond to Msgn1 expression despite the presence of E-boxes, thereby empirically validating the ChIP-seq analysis ( Fig. 6b ). The small peaks observed in Nrarp and Sprouty2 upstream sequences are of similar size to Dll1-2313 and were, therefore, not examined further. These results demonstrate that the Msgn1 ChIP-seq peaks examined are indeed cis -acting regulatory elements, and that Msgn1 functions as a strong transcriptional activator of Notch pathway genes. Msgn1 directly activates the segmentation clock gene Lfng We have shown that Msgn1 can bind and activate regulatory enhancers of the cyclic genes Dll1 , Maml3 , and Lfng , and that Msgn1 is required for the cyclic expression of Dll1 and Lfng in vivo . These results strongly suggest that Msgn1 is an important component of the segmentation clock. To address the mechanisms of Msgn1 function in the clock, we focused on understanding the transcriptional regulation of Lfng because the regulatory elements are well characterized in vivo [30] , [33] , [36] , and because Lfng is an important regulator of oscillating Notch activity [36] , [37] , [38] . Lfng transcription in the PSM is controlled by three separable, conserved elements termed blocks A, B and C [30] found within a 2.3-kb region upstream of the transcriptional start site [30] , [33] , [36] . An RBP-JK binding site (which confers Notch responsiveness) and two E-boxes identified within block A (Fringe Clock Element1 (ref. 33 ), regulate cyclic Lfng expression in the posterior PSM, whereas E and N-boxes in block B regulate expression in the anterior PSM [16] , [30] , [33] , [36] . Our genomic ChIP-seq studies showed that Msgn1 bound to both blocks A and B ( Fig. 7a ). Single gene ChIP–PCR assays in ESCs validated the ChIP-seq results, demonstrating that both blocks were highly enriched by F-Msgn1 ChIP ( Supplementary Fig. S5 ). Importantly, anti-Msgn1 antibodies ( Supplementary Fig. S6 ) detected endogenous Msgn1 bound to Lfng regulatory blocks A and B in PSM extracts but not in control extracts of the head ( Fig. 7b ). Electrophoretic mobility shift assays (EMSA) confirmed that Msgn1 protein indeed bound directly to E-box sequences found in the A and B block ( Supplementary Fig. S7 ), but not to the closely related N-boxes residing in block B. The results of the EMSA assays mirror the ChIP results, with Msgn1 generally showing greater binding affinity for block A than for block B, in both assays. Together, these results demonstrate that Lfng is a direct target gene of Msgn1, and that Msgn1 binds Lfng clock regulatory elements in vivo . The binding of Msgn1 to block A or to block B was sufficient to activate the expression of the luciferase reporter by 5- to 6-fold when either block was tested in isolation; however, Msgn1 alone did not strongly activate the reporter in the context of the longer 2.3-kb Lfng upstream region ( Fig. 7c ). This result argues that further activators are required to generate a robust transcriptional response, and that negative factors also regulate Lfng . The 2.3 kb construct did not respond well to activated Notch (NICD) either; however, the co-expression of Msgn1 and NICD resulted in a synergistic 7- to 15-fold induction of luciferase activity ( Fig. 7c,d ). This Msgn1–Notch synergism was mediated by block A because synergism was not observed with reporter constructs that lacked block A (see constructs B, C and BC), and was very strong (50- to 107-fold) when Msgn1 and NICD were co-expressed with the block A enhancer alone ( Fig. 7c,d ). Negative regulators presumably bind to blocks B and C because the Msgn1–Notch synergism is adversely affected by the presence of these blocks. Together, the data demonstrate that Msgn1 and the Notch signalling pathway regulate Lfng by binding directly to clock elements in block A to cooperatively activate transcription. Msgn1 activates the expression of multiple genes in the Notch pathway, including cyclic genes, however Msgn1 is not expressed periodically. How then are some Msgn1 target genes cyclically expressed, whereas others are not? In the case of the Msgn1–Notch target gene Lfng , oscillatory expression presumably arises from the dynamic activity of the Notch pathway. The Hairy enhancer-of-split ( Hes ) gene, Hes7 , is a periodically expressed Notch target gene and bHLH transcription factor that is required for somitogenesis and cyclic gene expression [39] , [40] . Hes7 has been proposed to function as the segmentation clock pacemaker as it operates in an autoinhibitory feedback loop and periodically represses Lfng transcription [28] . If Msgn1 is a major driver of clock gene expression and Hes7 is the pacemaker, then Hes7 should repress the activating activity of Msgn1 on Lfng . Indeed Hes7 completely repressed the activation of the full-length 2.3-kb Lfng enhancer by Msgn1 alone, or Msgn1 and Notch together ( Fig. 7d ). Examination of Hes7 activity on the isolated A or B blocks revealed that Hes7 repressed the activation of the block B enhancer by Msgn1 alone, but had no effect on the Msgn1-dependent activation of the block A cyclic enhancer. As Hes7-binding N-boxes are only found in block B, these results argue that Hes7 represses Lfng by binding to N-boxes. On the other hand, Hes7 does repress the combined activity of Msgn1 and Notch on the A block by 47% suggesting that at least some Hes7 repressor activity is N-box independent. Nevertheless, Msgn1 and Notch still function as powerful, synergistic activators of the Lfng block A clock enhancer, activating it 57-fold despite the presence of Hes7. The original clock and wavefront model first proposed that the sequential and repetitive formation of somites arises from a cellular oscillator (the clock) periodically interacting with a wavefront of rapid cell change that moves progressively down the embryonic anteroposterior axis [41] . The discovery of oscillating genes in the Notch, Wnt3a and Fgf signalling pathways, and the demonstration that Wnt3a/Fgf signalling gradients define the travelling wavefront or determination front, suggests that Wnt3a functions in both the clock and the wavefront during somitogenesis. In this study, we have shown that Wnt3a controls the clock and the wavefront through the activation of the direct target gene Msgn1 and that Msgn1 plays a pivotal role in the segmentation clock by functioning to coordinate the Wnt and Notch pathways. The expression of Wnt3a in the primitive streak (PS) and tailbud [7] , [20] establishes a descending posterior-to-anterior nuclear gradient in the PSM of the transcriptional coactivator β-catenin [17] . This β-catenin gradient is reflected in the graded expression of some direct Wnt3a/β-catenin target genes such as Axin2 (ref. 7 ). Axin2 appears to be universally responsive to Wnt/β-catenin signalling because it is expressed at multiple sites of Wnt activity in the embryo and adult, as well as in Wnt/β-catenin-dependent tumours and cancer cell lines [42] , [43] , [44] , [45] . In contrast, Msgn1 expression is restricted to the embryonic PSM and is less graded than Axin2 during early somitogenesis stages, displaying a more defined border in the anterior PSM. The absence of Msgn1 expression at other sites of Wnt activity argues that additional pathways are required for the activation of Msgn1 in the PSM. This is supported by the demonstration that Tbx6, which is co-expressed with Msgn1 in the PSM, cooperates with the Wnt3a/β-catenin pathway to directly regulate the Msgn1 promoter (this work; [23] ). The broad expression of Msgn1 throughout the posterior PSM, collapses into a weak gradient in the absence of Tbx6 , suggesting that a major function of Tbx6 is to convert the 'slope' of the Wnt3a gradient into a 'step' of Msgn1 expression that displays a defined anterior border. The anterior Msgn1 border lies immediately caudal to the seg-mental Mesp2 stripe and, therefore, marks the position of the determination front. Recent genetic studies have shown that the Wnt3a/β-catenin gradient regulates somitogenesis, at least in part, by positioning the determination front in the anterior PSM [8] , [17] . Our present work demonstrates that these same genetic manipulations of Wnt signalling that alter the determination front position, also correspondingly alter the position of the anterior boundary of Msgn1 expression. This boundary posteriorly regresses at the rate of one somite length during one period of somite formation [46] , indicating that the posterior-ward movement of the Msgn1 expression domain parallels the regression of the wavefront. Importantly, activation of Mesp2 and Ripply2 does not occur in Msgn1 −/− mutants ( Fig. 3 [19] ), suggesting that Msgn1 is required for posterior PSM progenitors to transition to anterior PSM fates and establish a segmental pre-pattern. Taken together, the data strongly argue that the Wnt3a/β-catenin gradient controls determination front activity through Msgn1 , and that the anterior border of Msgn1 has a key role in defining this activity. Recent work has affirmed the essential role that the Notch pathway has in the mammalian segmentation clock [9] . Wnt3a functions upstream of Notch to control cyclic gene expression in both the Wnt and Notch pathways, leading to the hypothesis that Wnt/β-catenin signalling drives the segmentation clock [7] . Studies of β-catenin mutants support this contention; however, the demonstration that Lfng continues to oscillate in the presence of a stabilized, non-cyclical form of β-catenin argues that β-catenin is not the clock pacemaker [8] , [17] . How, then does the Wnt3a/β-catenin pathway regulate Notch signalling and the segmentation clock? One way is through the direct activation of Dll1 [12] , [47] . We show here that Wnt3a, acting via Msgn1 , has a much broader role in Notch regulation, activating almost the entire Notch signalling pathway including cyclic target genes. Thus, Msgn1 is a master regulator of a Notch signalling gene expression program. Although Msgn1 is required for Notch target gene expression, the Wnt target genes Sp5 and Axin2 were upregulated in Msgn1 mutants. This expression is similar to the enhanced expression previously reported [19] for another Wnt3a target gene T/Brachyury [48] , suggesting that Msgn1 directly, or indirectly, represses some Wnt targets. The divergent response of Wnt and Notch targets suggest that Msgn1 functions to coordinate these pathways in the segmentation clock. Despite our proposal that it has a central role in the clock, Msgn1 is unlikely to function as the pacemaker because it is not expressed periodically. Our demonstration that Hes7 blocks the synergistic Msgn1-Notch activation of Lfng is consistent with previous suggestions that Hes7 is the pacemaker [28] . We suggest that cyclic gene expression in the Notch pathway requires two primary regulatory components: an activator, arising from the combined activity of Msgn1 and the Notch signalling pathway, and a short-lived periodic repressor, Hes7, which functions in an autoinhibitory feedback loop to periodically repress Hes7 and Lfng ( Fig. 8 ). Although it is well known that the Fgf pathway is also required for cyclic gene expression and for the proper expression of Msgn1 (ref. 10 ), the precise mechanisms remain unclear. 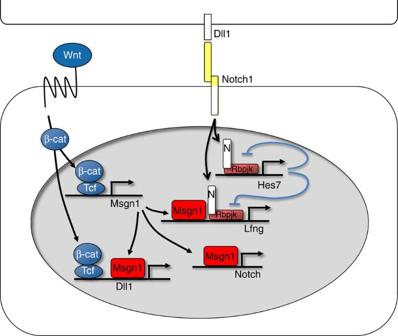Figure 8: Schematic model of the regulation of Notch pathway genes and the segmentation clock by the Wnt3a/β-catenin target geneMsgn1. The Wnt3a/β-catenin pathway directly activatesMsgn1andDll1. Msgn1 binds directly to regulatory enhancers to activate gene expression in the PSM. Direct activation ofDll1by Msgn1 establishes a feed-forward loop that ensures strong activation ofDll1by Wnt signals. Msgn1 synergizes with activated Notch to activateLfng. The Notch target, and clock pacemaker, Hes7, functions in an autoinhibitory feedback loop (blue lines) to periodically repress its own expression, and that ofLfng, thereby driving the oscillating segmentation clock. The ability of Msgn1 to bridge the Wnt and Notch pathways suggests an explanation for the antiphase nature of Wnt and Notch clock gene expression7. Active Wnt signalling initiates the expression ofMsgn1and cyclic Wnt target genes such asAxin2, whereas a phase-lag, to allow for the transcription and translation ofMsgn1and the activation of Msgn1-Notch target genes, leads to the delayed expression ofLfng. For simplicity, several target genes, gene products, and regulatory interactions are not shown. Figure 8: Schematic model of the regulation of Notch pathway genes and the segmentation clock by the Wnt3a/β-catenin target gene Msgn1 . The Wnt3a/β-catenin pathway directly activates Msgn1 and Dll1 . Msgn1 binds directly to regulatory enhancers to activate gene expression in the PSM. Direct activation of Dll1 by Msgn1 establishes a feed-forward loop that ensures strong activation of Dll1 by Wnt signals. Msgn1 synergizes with activated Notch to activate Lfng . The Notch target, and clock pacemaker, Hes7, functions in an autoinhibitory feedback loop (blue lines) to periodically repress its own expression, and that of Lfng , thereby driving the oscillating segmentation clock. The ability of Msgn1 to bridge the Wnt and Notch pathways suggests an explanation for the antiphase nature of Wnt and Notch clock gene expression [7] . Active Wnt signalling initiates the expression of Msgn1 and cyclic Wnt target genes such as Axin2 , whereas a phase-lag, to allow for the transcription and translation of Msgn1 and the activation of Msgn1-Notch target genes, leads to the delayed expression of Lfng . For simplicity, several target genes, gene products, and regulatory interactions are not shown. Full size image Interactions between the Notch and Wnt pathways are known to regulate the maintenance of stem cells, including hematopoietic and gastrointestinal stem cells [49] , [50] , [51] . This raises the intriguing possibility that a similar relationship between the Wnt and Notch pathways could regulate mesodermal stem cells in the segmenting embryo. Indeed, we know that Msgn1 controls the maturation of these mesodermal progenitors because they accumulate as an undifferentiated mass in the tailbud of Msgn1 −/− embryos [19] and display impaired anterior-ward migration and epithelial-mesenchymal transitions. Because Wnt3a regulates the same processes, it is possible that Wnt3a regulates mesodermal stem cell homeostasis, migration, epithelial-mesenchymal transitions, and positional information through Msgn1 . The identification of the interacting proteins, and the genomic targets, of Msgn1 will greatly assist in our understanding of how Wnt signals regulate such numerous and diverse processes. Mice Ctnnb1 tm2Kem mice were purchased from the Jackson Labs. The Wnt3a (ref. 20 ), Mesogenin1 (ref. 19 ), Ctnnb1 lox(ex3) (ref. 52 ), Tbx6 (ref. 24 and T-cre mice (ref. 53 ) were obtained from the originating labs. Transgenic mice were generated in the Transgenic Core Facility, NCI-Frederick, by pronuclear injection following standard procedures. All animal experiments were performed in accordance with the guidelines established by the NCI-Frederick Animal Care and Use Committee. Whole-mount in situ hybridization Whole-mount in situ hybridization (WISH) and section in situ hybridization (ISH) were performed as described [14] . Unless indicated otherwise, at least four mutant embryos were examined for each probe, and all yielded similar results. ES cell culture and differentiation Serum independent GFP-Bry embryonic stem cells (ESC) were maintained and differentiated into mesoderm as described [22] . Recombinant Wnt3a protein (R&D Systems) was added to embryoid bodies on D2 of differentiation and cells were collected for RNA extraction 48 h later. The Msgn1 ORF with amino-terminal 1× or 3× FLAG tags were cloned into p2lox targeting vector, and site-specific recombination was accomplished by inducing A2lox.cre ESCs [31] with Doxycycline (Dox) 24 h before electroporation with the P2lox-FLAG-Msgn1 vector. For EB differentiation, ESC were plated on 10 cm Petri dishes at a density of 2.5 million cells per plate in 15 ml of DMEM, 10% FBS, NEAA, Pen/Strep, 2-Mercaptoethanol and 50 μg ml −1 ascorbic acid (Sigma). After 2 days of differentiation, EBs were then transferred to 6-well ultra low attachment dishes (Corning) and expression of FLAG-Msgn1 was induced using 1 μg per ml Dox. Samples were collected at 12-h interval up to 48-h. The same EB differentiation protocols were used for transcriptional profiling and ChIP-seq assays. Gene expression profiling Gene expression profiling on microdissected node and primitive streak regions of E7.75–E8 wildtype and Wnt3a −/− embryos was performed as described [8] . For ESC expression profiling, total RNA was isolated using RNeasy mini kit (Qiagen) from EBs treated with and without doxycycline at 12-, 24- and 48-h time intervals according to manufacturer's instructions. Protocols for synthesis of complementary DNA and antisense RNA were performed using the Affymetrix Genechip 3′ IVT Express kit (Affymetrix) according to manufacturer's recommendations. Statistical analysis was performed on probe-intensity level data (CEL files) using Genespring GX10 (Agilent) and BRB-ArrayTools Version.3.2 software. Initial filtering and preprocessing, including background correction, quantile normalization and summarization, was performed using the robust multi-array analysis algorithm. Statistical analyses were performed using an unpaired t -test at P ≤0.05 on genes displaying a fold change of 1.5 or greater. The mean-normalized intensity values (log 2 values) and standard deviation for each gene were calculated and plotted. Protein studies Polyclonal mouse antibodies against Msgn1 protein were made by A&G Precision antibody (Columbia) using a cocktail of peptides CWKSRARPLELVQESP, CDLLNSSGREPRPQSV, CSHEAAGLVELDYS conjugated to KLH antigen. Chromatin immunoprecipitation assays ChIP of EBs: 36 h after Dox induction, EBs were fixed in 1% formaldehyde solution for 15 min and quenched with 0.125 M Glycine. Cells were lysed with lysis buffer and chromatin was sheared to an average length of 300–500 bp as described [54] . Protein DNA complexes were immunoprecipitated using anti-FlagM5 antibody or corresponding isotype. Crosslinks were reversed and DNA was extracted with phenol:chloroform and purified by ethanol precipitation. The Chromatin immunoprecipitation-sequencing (ChIP-Seq) approach was performed by Genpathway (San Diego, California) [55] . Briefly EBs were fixed and quenched as described above, and flash frozen. The nuclei were extracted, sonicated and precleared with Staph A cells (Pansorbin, Calbiochem) before incubation with anti-Flag M2 antibody (Sigma). Samples were incubated with prepared Staph A cells to extract antibody-chromatin complexes, followed by washing and elution. Precipitated DNA fragments were released and purified. ChIP DNA fragments associated with FLAG-Msgn1 were amplified using the Illumina ChIP-Seq DNA sample prep kit (Illumina). DNA libraries were sequenced on a Genome Analyser II by Illumina Sequencing Services. 35-nt sequence reads were mapped to the genome using the Eland algorithm. The 35 bp sequences were extended in silico at the 3′ end up to 110 bp, which is the average DNA fragment length after shearing. The resulting histograms were stored in BAR (Binary Analysis Results) files. For each BAR file, intervals were calculated and compiled into BED files (Browser Extensible Data) for viewing in the UCSC genome browser. Enriched intervals, referred to as peak values, were determined by applying a threshold P -value cut-off of 10e−5 and a false discovery rate (FDR) of 2.35%. BAR files were uploaded to the Integrated Genome Browser (IGB-Affymetrix) for extensive analysis. ChIP of embryo tissues: About 60 PSMs and 25 heads from E9.5 stage embryos were collected and fixed overnight in 4% PFA at 4 °C and dehydrated in methanol series [56] . On the day of the CHIP assay, PSM and head tissues were rehydrated, cross-linked with 1% formaldehyde for 15 min at room temperature and quenched with 0.125 M glycine. Tissues were washed 2× with ice-cold PBS, resuspended in lysis buffer LB1 [54] and disrupted by passing through 26 3/8 gauge needle. Pellets in lysis buffer LB3 were sonicated using Branson Sonifer450 and lysates were pre-cleared for 15 min at 4 °C with 20 μl proteinG dynal beads (Invitrogen) pre-blocked with 0.5% BSA in PBS and 1 mg ml −1 sonicated salmon sperm DNA (Ambion). Equal amounts of lysates were immunoprecipitated with anti-Msgn1 ascites or control ascites (Clone NS-1; Sigma). Half-embryo explant cultures Half-embryo explant cultures were done as described [8] . PSM explants of wild type and Msgn1 −/− embryos were dissected at E8.25–E8.5 and manually bisected along the midline. The left half of the embryo was immediately fixed in 4% PFA, while the right half was cultured at 37° C for 60 or 90 min in DMEM with 10% FBS supplemented with 10 ng per ml bFGF (R and D Systems) before fixation. Expression constructs and luciferase reporter assays Reporter constructs of 1 kb Msgn1 promoter and mutant version of 3 TCF/LEF binding sites were generated in pGL4.10(luc2) vector (Promega). For generating transgenic mice, the hsp68 minimal promoter was replaced with the wildtype and TCF/LEF mutated 1 kb Msgn1 promoter followed by lacZ and SV40polyA signal in pASShsp68-lacZ-pA vector. The luciferase reporter construct containing the 2.3 kb Lunatic-fringe cyclic enhancer [30] , Lfng enhancer deletion constructs, and positively identified CHIP seq peaks were generated in the pGL4.23 [ minp-luc2 ] vector (Promega). HEK293T cells or NIH 3T3 cells were seeded at 0.25×10 5 cells per well in 24 well plates and cultured for 18 h. A total of 500 ng of DNA containing the reporter plasmids (200 ng) and empty luciferase vectors were co-transfected with or without expression vectors pSG5-T-VP16 (50 ng), pcDNA-Tbx6-VP16 (50 ng), ΔN-βcatenin-myc (50 ng), pCS2-Myc-Msgn1 (100 ng), CMV-3xFlag-Mesp2 (100 ng), and pCS2-NICD-Venus (50 ng), CMV-3xFlag-Hes7 (100 ng) using Lipofectamine 2000 (Invitrogen). Equivalent amounts of DNA were achieved with pcDNA3 or pCS2 vector. Cells were lysed 40 h after transfection and luciferase activity was measured using the Dual Luciferase Assay Kit (Promega) as per manufacturers recommendations. In each condition, 5 ng of pGL4.74 [hRluc/TK] Vector (Promega) was used as an internal control to normalize for transfection efficiency. Fold change was calculated as a ratio of the luciferase vector containing Msgn1 or Lfng regulatory elements relative to empty luciferase vector for identical experimental conditions, normalized to a control condition minus expression vectors. The reported values are from one experiment but are representative of at least three independent experiments. Electrophoretic mobility shift assay Lef1 and Myc-Msgn1 proteins were made using the TNT Reticulocyte Lysate System (Promega) in vitro . Double stranded DNA oligonucleotides were end labelled with DIG-ddUTP and protein-DNA complexes were analysed using the DIG Gel Shift Assay Kit (Roche) according to manufacturer's instructions. Reverse transcription and qPCR 1 μg of RNA was Dnase1 treated and first-strand cDNA was synthesized using oligo dT and superscript III reverse transcriptase (Invitrogen) or iScript cDNA synthesis kit (Roche) according to manufacturers instructions. qPCR analysis was used to quantitate cDNAs using CFX96 Real-Time PCR Detection System (Bio-Rad) and Fast Start Universal SYBR Green Master (Roche). For the qPCR results shown in Figure 1h , Taqman gene expression assays were performed (Mm00490407_S1) using Taqman universal PCR Master Mix (Applied Biosystems) according to manufacturer's recommendations. Gapdh expression was used to normalize Msgn1 expression values. The specificity of all primers was monitored by electrophoresis of the amplicons on agarose gels. The mean expression values obtained for each gene were normalized to GAPDH (ΔΔC (t) method) and to the expression in undifferentiated ES cells. For normalization of CHIP-qPCR analysis, first percent input method was used to calculate from the obtained Ct values and was further normalized to the values obtained in the control ascites to obtain the fold change values. All CHIP and qPCR experiments were done in triplicates. See Supplementary Table S2 for oligonucleotide sequences used in EMSA and qPCR assays. Accession codes: The microarray data have been deposited in the GEO database under accession code GSE29848 and GSE29995 . How to cite this article: Chalamalasetty, R. B. et al . The Wnt3a/β-catenin target gene Mesogenin1 controls the segmentation clock by activating a Notch signalling program. Nat. Commun. 2:390 doi: 10.1038/ncomms1381 (2011).